NiPS3ultrathin nanosheets as versatile platform advancing highly active photocatalytic H2production High-performance and low-cost photocatalysts play the key role in achieving the large-scale solar hydrogen production. In this work, we report a liquid-exfoliation approach to prepare NiPS 3 ultrathin nanosheets as a versatile platform to greatly improve the light-induced hydrogen production on various photocatalysts, including TiO 2 , CdS, In 2 ZnS 4 and C 3 N 4 . The superb visible-light-induced hydrogen production rate (13,600 μmol h −1 g −1 ) is achieved on NiPS 3 /CdS hetero-junction with the highest improvement factor (~1,667%) compared with that of pure CdS. This significantly better performance is attributed to the strongly correlated NiPS 3 /CdS interface assuring efficient electron-hole dissociation/transport, as well as abundant atomic-level edge P/S sites and activated basal S sites on NiPS 3 ultrathin nanosheets advancing hydrogen evolution. These findings are revealed by the state-of-art characterizations and theoretical computations. Our work for the first time demonstrates the great potential of metal phosphorous chalcogenide as a general platform to tremendously raise the performance of different photocatalysts. The enormous consumption of non-renewable fossil fuels has led to the global energy shortage, environmental pollution and climate change. Therefore, seeking renewable, clean and carbon-free energy sources is of paramount importance. Solar hydrogen (H 2 ) production via photocatalytic water splitting is considered a promising, inexpensive and environmentally benign technique to generate green H 2 fuel using sunlight [1] , [2] , [3] , [4] , [5] , [6] , [7] , [8] , [9] , [10] , [11] , [12] , [13] , [14] , [15] , [16] , [17] , [18] , [19] , [20] , [21] , [22] , [23] , [24] , [25] , [26] , [27] , [28] , [29] , [30] , [31] , [32] , [33] , [34] , [35] , [36] . However, the large-scale application of this photocatalytic process is severely restricted by the low efficiency, poor stability and the high price of photocatalysts developed to date. Hence, seeking highly-active, robust and cheap photocatalysts is of great significance for realizing industrial-scale solar H 2 generation [1] , [2] , [3] , [4] , [5] , [6] , [7] , [8] , [9] , [10] , [11] , [12] , [13] , [14] , [15] , [16] , [17] , [18] , [19] , [20] , [21] , [22] , [23] , [24] , [25] , [26] , [27] , [28] , [29] , [30] , [31] , [32] , [33] , [34] , [35] , [36] . Rational design and preparation of high-performance photocatalysts require not only the atomic-level understanding of the structure/composition–activity relationship [9] , [10] , [23] , [37] , [38] , [39] , [40] , [41] , [42] but also the precise and insightful apprehension of the kinetics and thermodynamics of photo-generated electrons and holes in photocatalysts [5] , [12] , [43] , [44] , [45] , [46] , [47] , [48] , [49] Merging the atomic-resolution aberration-corrected scanning transmission electron microscopy (AC-STEM) and theoretical computations could provide the atomic-level knowledge about the structure/composition-activity correlation for photocatalysts [9] , [10] , [23] , [37] , [38] , [39] , [40] , [41] , [42] . Particularly, various atomic-level reactive sites, e.g., single atoms [9] , [10] , [23] , [37] , [42] , edge sites [41] and defects [38] , [39] , [40] , [42] , present in photocatalysts can be accurately revealed by the aforementioned approach. On the other hand, the separation/migration of photogenerated electrons and holes serve a pivotal role in determining the overall photocatalytic performance [1] , [2] , [3] , [4] , [5] , [6] , [7] , [8] , [9] , [10] , [11] , [12] , [13] , [14] , [15] , [16] , [17] , [18] , [19] , [20] , [21] , [22] , [23] , [24] , [25] , [26] , [27] , [28] , [29] , [30] , [31] , [32] , [33] , [34] , [35] , [36] , [43] , [44] , [45] , [46] , [47] , [48] , [49] . Thus, it is essential to adopt various advanced characterizations, e.g., ultrafast transient absorption spectroscopy (TAS), transient-state surface photovoltage (SPV) spectroscopy, transient-state photoluminescence (PL) spectroscopy and in situ X-ray photoelectron spectroscopy (XPS), for time-resolved study on the kinetics and thermodynamics of photogenerated electrons/holes in the bulk and, especially, on the surface of photocatalysts. Furthermore, it is of great importance to combine the above two strategies for simultaneous assessment of both the atomic-level structure/composition-performance relationship and the time-resolved charge-carrier separation/transfer mechanism for photocatalysts. Recently, two-dimensional (2D) transitional metal phosphorous chalcogenides (MPC x ) (M = Cr, Mn, Fe, Co, Ni, Zn, Ga, Cd, Sn and Bi; C = S, Se and Te) have attracted increasing attention in catalysis [50] , [51] , [52] , [53] , [54] , [55] , [56] , [57] , [58] , [59] , [60] , [61] , [62] , (opto)electronics [63] , [64] and sensing [65] owing to the distinct physicochemical properties. Nevertheless, this large group of materials is rarely applied in photocatalysis. This group of materials, due to their unique properties, is regarded as a potentially excellent platform for enhancing photocatalysis, which is ascribed to the following features: (1) ultrathin thickness favouring the dissociation of photogenerated electrons/holes, and transport to the surface; (2) large surface area facilitating the formation of strong interfacial electronic coupling with other materials; (3) abundant surface reactive sites promoting the redox catalytic reactions on the surface, and (4) thickness-dependent band gap width benefiting the flexible adjustment of electronic band structures for balancing light absorption and redox abilities of electrons/holes. To date, several experimental [50] , [51] , [52] , [53] , [54] , [55] , [56] and computational [61] , [62] works on 2D MPC x materials in photocatalysis have been reported. For instance, Wang et al. [52] reported that 2D NiPS 3 nanosheets achieved the photocatalytic H 2 -production rates of ~26.4 and 74.67 μmol h −1 g −1 from pure water and Na 2 S/Na 2 SO 3 aqueous solution, respectively, under xenon light irradiation. Additionally, Barua et al. [53] reported the photocatalytic H 2 -production activity of 2600 μmol h −1 g −1 on Eosin Y-sensitized NiPS 3 nanosheets in triethanolamine aqueous solution using a xenon lamp. Furthermore, FePS 3 quantum sheets were synthesized to attain the photocatalytic H 2 -production rate of 290 μmol h −1 g −1 in triethanolamine aqueous solution using xenon light [51] . Moreover, theoretical computations were conducted to calculate the band gaps and band edge positions of MPS 3 (M = Fe, Mn, Ni, Cd and Zn) and MPSe 3 (M = Fe and Mn) monolayers [62] . These MPS 3 /MPSe 3 monolayers were found to be good candidates for photocatalytic water splitting. Nevertheless, the application of MPC x family as a general platform to greatly enhance the light-induced H 2 -production performance on various semiconductor photocatalysts, e.g., metal oxides, metal sulfides and metal-free nitrides, is not reported to date. Here for the first time, we report a new liquid-exfoliation approach to acquire 2D MPC x , NiPS 3 ultrathin nanosheets (UNSs), as a versatile platform to apparently enhance the photocatalytic H 2 -production rates of metal oxide (TiO 2 ), metal sulfides (CdS and In 2 ZnS 4 ), and metal-free nitride (C 3 N 4 ), respectively. Among them, the NiPS 3 /CdS heterojunction exhibits the largest photocatalytic H 2 -production rate of 13,600 μmol h −1 g −1 with the highest enhancement factor of ~1667% compared to CdS alone. The increased photocatalytic H 2 production arises from the intimate electronic coupling promoting the interfacial charge separation/migration and the abundant atomic-level P/S edge sites together with activated S basal sites of NiPS 3 boosting H 2 evolution reaction. These findings are supported by both theoretical computations and state-of-art characterizations, which include atomic-resolution AC-STEM, electron energy loss (EELS) spectroscopy, synchrotron-based X-ray absorption near edge spectroscopy (XANES), in situ XPS, transient-state SPV spectroscopy, ultrafast TAS, transient-state PL spectroscopy and light-irradiated contact potential difference (CPD) test. This study further confirms the generality of NiPS 3 UNSs in conjunction with the other semiconductor photocatalysts, e.g., TiO 2 , In 2 ZnS 4 and C 3 N 4 , toward elevated photocatalytic H 2 production. Our work not only demonstrates the great potential of this large MPC x group in the photocatalysis field but more importantly, paves avenues for the rational design and preparation of high-performance photocatalysts via merging the advanced characterizations and theoretical calculations. Theoretical prediction, synthesis, characterization and application of 2D NiPS 3 We selected NiPS 3 from a series of transitional metal phosphorous chalcogenides (MPC x ) (M = Cr, Mn, Fe, Co, Ni, Zn, Ga, Cd, Sn and Bi; C = S, Se and Te) and predicted the potential properties via density functional theory (DFT) based computations. 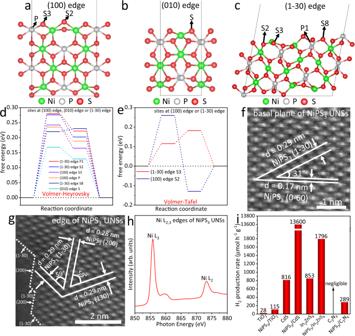Fig. 1: Theoretical prediction, characterization and application of NiPS3UNSs. aActive P, S2 and S3 sites for HER at (100) edge of NiPS3monolayer.bActive S site for HER at (010) edge of NiPS3monolayer.cActive P1, S2, S3 and S8 sites for HER at (1–30) edge of NiPS3monolayer.dGibbs free energy diagrams for HER following the Volmer–Heyrovsky pathway on the active sites at (100) edge, (010) edge or (1−30) edge of NiPS3monolayer.eGibbs free energy diagrams for HER following the Volmer–Tafel pathway on the active sites at (100) or (1−30) edge of NiPS3monolayer. Atomic-resolution HAADF-STEM images forfbasal plane andgedge of NiPS3UNSs. Synchrotron-based XANEShNi L2,3edges of NiPS3UNSs.iPhotocatalytic H2-production rates for TiO2, NiPS3/TiO2, CdS, NiPS3/CdS, In2ZnS4, NiPS3/In2ZnS4, C3N4and NiPS3/C3N4in ~17.0 vol% triethanolamine aqueous solution. Among them, TiO2and NiPS3/TiO2were excited by xenon light without cut-off filter. CdS, NiPS3/CdS, In2ZnS4, NiPS3/In2ZnS4, C3N4and NiPS3/C3N4were excited by visible-light irradiation (λ> 400 nm). All the Gibbs free energies were calculated considering the solvation effect in 17 vol% triethanolamine aqueous solution. We made this selection based on the previous experimental results as summarized in Supplementary Table 1 . As shown in Supplementary Table 1 , among all the reported MPS x and MPSe x , NiPS 3 shows the lowest overpotential (193 mV) for electrochemical hydrogen evolution reaction (HER) in the alkaline solution, as the current density reaches −10 mA cm −2 . Besides, considering that MPTe x is rarely reported for photocatalytic/electrocatalytic hydrogen (H 2 ) evolution, we decide to select NiPS 3 and study its HER ability using DFT-based calculations. In this work, we focus on the HER activity to explore whether NiPS 3 can serve as a versatile platform promoting photocatalytic H 2 production. Generally, a three-state diagram, which consists of an initial state H + + e − , an intermediate adsorbed H*, and a final product ½H 2 , is utilized to summarize the whole HER process. The Gibbs free energy of the intermediate state, |Δ G H* |, is considered a major indicator for the HER activity on different types of catalysts. The most desirable value of |Δ G H* | is zero. For instance, the well-known HER catalyst with excellent activity, Pt, exhibits a near-zero value of Δ G H* ≈ −0.09 eV. As a result, we apply DFT-based computations to calculate the Δ G H* values for the sites at the basal plane and edge of NiPS 3 monolayer. Twenty-four possible HER active sites on the basal plane (Supplementary Fig. 1a–c ), (100) edge (Supplementary Fig. 1d–f ), (010) edge (Supplementary Fig. 1g–i ) and (1–30) edge (Supplementary Figs. 2a–f and 3a–i ) of NiPS 3 monolayer were studied to predict the most active sites for HER. Accordingly, the HER free energy diagrams via either the Volmer–Heyrovsky pathway (Supplementary Figs. 1b, e, h , 2b, e and 3b, e, h ) or the Volmer–Tafel pathway (Supplementary Figs. 1c, f, i , 2c, f and 3c, f, i ) were acquired to disclose the reaction mechanism. The corresponding Δ G H* values via either Volmer–Heyrovsky or Volmer–Tafel pathway are displayed in Supplementary Tables 2 – 6 . All the above theoretical calculations were performed considering the solvation effect in 17 vol% triethanolamine aqueous solution, in which the HER will occur. Among these 24 HER active sites, 8 most active sites for HER are displayed in Fig. 1a–c , which are P, S2 and S3 sites at (100) edge, S site at (010) edge together with P1, S2, S3 and S8 sites at (1–30) edge of NiPS 3 monolayer. Furthermore, based on the Δ G H* values of these 8 active sites (Supplementary Tables 3 – 6 ), the P and S3 sites at (100) edge, S site at (010) edge together with P1, S2 and S8 sites at (1–30) edge follow the Volmer-Heyrovsky pathway (Fig. 1d ); while the S2 site at (100) edge and S3 site at (1–30) edge follow the Volmer-Tafel pathway (Fig. 1e ). Among the other 16 sites of NiPS 3 monolayer, S4, S5 and S7 sites at (1–30) edge show the small │Δ G H* │values for Volmer step owing to the edge effect (Supplementary Table 6 ). However, they are not deemed as effective active sites because of the high free energy change for the second step of H 2 formation (Supplementary Table 6 ). Overall, the aforementioned DFT-based computations reveal the excellent HER activities on specific P and S edge sites of NiPS 3 monolayer. In comparison, the basal plane sites and Ni edge sites of NiPS 3 monolayer are not considered the active sites for HER. 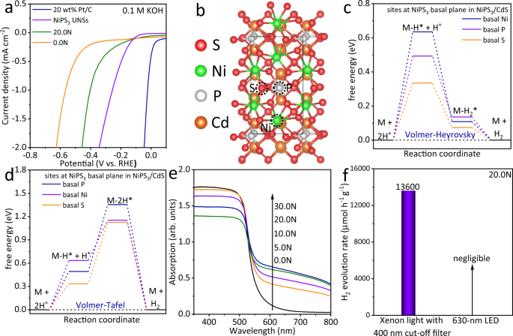Fig. 6: Surface catalytic reactions and light absorption of NiPS3/CdS system. aElectrochemical HER activities in 0.1 M KOH aqueous solution for 0.0N, 20.0N, NiPS3UNSs and 20 wt% Pt/C.btop-view atomic structure of NiPS3/CdS showing the Ni, P and S basal sites.cThe calculated free energy diagrams of HER following the Volmer-Heyrovsky pathway on the Ni, P and S sites of NiPS3basal plane in NiPS3/CdS system.dThe calculated free energy diagrams of HER following the Volmer-Tafel pathway on the Ni, P and S sites of NiPS3basal plane in NiPS3/CdS system.eUV-Vis diffuse reflectance spectra of 0.0N, 5.0N, 10.0N, 20.0N and 30.0N.fPhotocatalytic H2-production rates measured for 20.0N in ~17.0 vol% triethanolamine aqueous solution with xenon light irradiation (λ> 400 nm) and 630-nm LED, respectively. All the Gibbs free energy calculations were conducted considering the solvation effect in 17 vol% triethanolamine aqueous solution. On the other hand, 2D NiPS 3 also possesses the well-known advantages of ultrathin thickness and large surface area. These properties not only facilitate the efficient bulk-to-surface charge carrier migration but also enhance electronic interaction with other materials for rapid interfacial charge carrier transport and optimized catalytic activities. Fig. 1: Theoretical prediction, characterization and application of NiPS 3 UNSs. 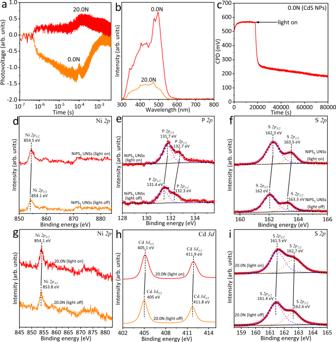a Active P, S2 and S3 sites for HER at (100) edge of NiPS 3 monolayer. Fig. 5: Charge carrier kinetics in NiPS3/CdS system. aTransient-state andbsteady-state SPV spectra of 0.0N and 20.0N.cCPD test of 0.0N in the dark and under light irradiation. High-resolution XPS spectra ofdNi2p,eP2pandfS2pof NiPS3UNSs with the light on and off, respectively. High-resolution XPS spectra ofgNi2p,hCd3dandiS2pof 20.0N with the light on and off, respectively. 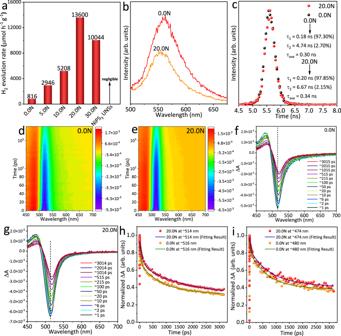b Active S site for HER at (010) edge of NiPS 3 monolayer. c Active P1, S2, S3 and S8 sites for HER at (1–30) edge of NiPS 3 monolayer. Fig. 4: Photocatalytic H2-production activities and charge carrier kinetics of NiPS3/CdS system. aPhotocatalytic H2-production rates of 0.0N, 5.0N, 10.0N, 20.0N, 30.0N and NiPS3UNSs in ~17.0 vol% triethanolamine aqueous solution using visible-light illumination (λ> 400 nm).bSteady-state andctransient-state PL spectra of 0.0N and 20.0N.cInset shows the fitting charge lifetimes for 0.0N and 20.0N. 2D pseudocolor TA spectra ofd0.0N ande20.0N in ethanol solution after the excitation with a 400 nm laser pulse. The TA spectra off0.0N andg20.0N at different pump-probe delay time.hNormalized decay kinetics and fitting lines for 0.0N and 20.0N taken through the GSB peaks at ~516 and ~514 nm, respectively.iNormalized decay kinetics and fitting lines for 0.0N and 20.0N taken through the ESA peaks at ~480 and ~474 nm, respectively. d Gibbs free energy diagrams for HER following the Volmer–Heyrovsky pathway on the active sites at (100) edge, (010) edge or (1−30) edge of NiPS 3 monolayer. e Gibbs free energy diagrams for HER following the Volmer–Tafel pathway on the active sites at (100) or (1−30) edge of NiPS 3 monolayer. Atomic-resolution HAADF-STEM images for f basal plane and g edge of NiPS 3 UNSs. Synchrotron-based XANES h Ni L 2,3 edges of NiPS 3 UNSs. i Photocatalytic H 2 -production rates for TiO 2 , NiPS 3 /TiO 2 , CdS, NiPS 3 /CdS, In 2 ZnS 4 , NiPS 3 /In 2 ZnS 4 , C 3 N 4 and NiPS 3 /C 3 N 4 in ~17.0 vol% triethanolamine aqueous solution. Among them, TiO 2 and NiPS 3 /TiO 2 were excited by xenon light without cut-off filter. CdS, NiPS 3 /CdS, In 2 ZnS 4 , NiPS 3 /In 2 ZnS 4 , C 3 N 4 and NiPS 3 /C 3 N 4 were excited by visible-light irradiation ( λ > 400 nm). All the Gibbs free energies were calculated considering the solvation effect in 17 vol% triethanolamine aqueous solution. Full size image Thus, we developed a new and facile liquid exfoliation procedure (see methods) to obtain the NiPS 3 ultrathin nanosheets (UNSs) in ethanol. The transmission electron microscopy (TEM) image in Supplementary Fig. 4a shows NiPS 3 UNSs with lateral sizes of ~216–263 nm. The high-resolution (HR)TEM image of NiPS 3 UNSs (Supplementary Fig. 4b ) shows the lattice spacing value of 0.17 nm, in accordance with the (0−60) facet of monoclinic NiPS 3 . The energy dispersive X-ray spectroscopy (EDX) pattern of NiPS 3 UNSs (Supplementary Fig. 4c ) shows the presence of Ni, P and S, in agreement with the TEM and HRTEM results. Moreover, the high-angle annular dark field scanning transmission electron microscopy (HAADF-STEM) image (Supplementary Fig. 5a ) and the corresponding elemental mapping images of Ni (Supplementary Fig. 5b ), S (Supplementary Fig. 5c ) and P (Supplementary Fig. 5d ) again confirm the successful preparation of NiPS 3 UNSs. The atomic-resolution HAADF-STEM image (Fig. 1f ) of the basal plane for NiPS 3 UNSs shows two lattice spacing values of 0.29 and 0.17 nm, together with an angle of 31°. These two crystal planes, respectively, correspond to the (1−30) and (0−60) planes of monoclinic NiPS 3 . Additionally, three lattice spacing values of 0.29, 0.28 and 0.29 nm together with two angles of 59° and 59° are observed in Fig. 1g . These three crystal planes are assigned to the (1−30), (200) and (130) planes of monoclinic NiPS 3 , respectively. Furthermore, many steps along the (1−30) and (200) edges of NiPS 3 UNSs can be observed in Fig. 1g , indicating the existence of many P and S active sites at the edges of NiPS 3 UNSs. This implies the high activity of NiPS 3 UNSs toward HER. The atomic force microscopy (AFM) image of NiPS 3 UNSs (Supplementary Fig. 6a ) shows the UNS morphology with lateral sizes of ~157–480 nm. The corresponding height profile of NiPS 3 UNSs (Supplementary Fig. 6b ) exhibits a thickness of ~3.16 nm, verifying the ultrathin thickness. Such a thickness (~3.16 nm) corresponds to 3 or 4 atomic layers of NiPS 3 based on the single-layer thickness of ~0.8–1.1 nm [63] . The high-resolution XPS spectra of Ni 2p (Supplementary Fig. 7a ), P 2p (Supplementary Fig. 7b ) and S 2p (Supplementary Fig. 7c ) of NiPS 3 UNSs are in accordance with those reported elsewhere [60] . Moreover, the synchrotron-based X-ray absorption near edge spectroscopy (XANES) Ni L 2,3 edges for NiPS 3 UNSs are displayed in Fig. 1h . The Raman spectrum of NiPS 3 UNSs (Supplementary Fig. 8a ) exhibits the presence of E (2) g , A (1) 1g , A (2) 1g and A (3) 1g modes, in agreement with the prior report [60] . Moreover, the UV-Vis absorption spectrum of NiPS 3 UNSs (Supplementary Fig. 8b ) exhibits the absorption edge at 873 nm, suggesting the narrow band gap width (E) of 1.42 eV. The picture of NiPS 3 UNSs ethanol solution (Supplementary Fig. 8b inset) shows the typical Tyndall effect, indicating the formation of a homogeneous dispersion of NiPS 3 UNSs in ethanol. To explore the potential application of the as-prepared NiPS 3 UNSs in photocatalysis, we first investigate the detailed electronic band structure of NiPS 3 UNSs. The flat band potential of NiPS 3 UNSs is −0.58 V vs. Ag/AgCl electrode (Supplementary Fig. 9a ). Thus, the Fermi level ( E F ) of NiPS 3 UNSs is 0.05 V vs. standard hydrogen electrode (SHE). The XPS valence band (VB) spectrum of NiPS 3 UNSs (Supplementary Fig. 9b ) indicates that the VB edge potential of NiPS 3 UNSs is 0.81 V vs. E F of NiPS 3 UNSs. Hence, the VB edge potential of NiPS 3 UNSs is 0.86 V vs. SHE. As a result, the conduction band (CB) edge potential of NiPS 3 UNSs is −0.56 V vs. SHE, based on the band gap of NiPS 3 UNSs ( E = 1.42 eV). The electronic band structure of NiPS 3 UNSs is displayed in Supplementary Fig. 10 . The CB edge potential of NiPS 3 UNSs (−0.56 V vs. SHE) is much more negative than the HER potential (0.0 V vs. SHE). However, the VB edge potential of NiPS 3 UNSs (0.86 V vs. SHE) is not sufficiently positive for the oxygen evolution reaction (1.23 V vs. SHE). These results reveal the strong reduction ability of photogenerated electrons and weak oxidation capacity of photogenerated holes in NiPS 3 UNSs. On the other hand, the narrow band gap ( E = 1.42 eV) of NiPS 3 UNSs implies a wide light-responsive range (up to 873 nm) and excellent electronic conductivity. Nevertheless, the poor oxidation ability of photogenerated holes in NiPS 3 UNSs renders it more suitable to be merged with other semiconductor photocatalysts supplying strongly oxidative photogenerated holes rather than being used alone. Therefore, interface engineering was applied to combine NiPS 3 UNSs with other semiconductor photocatalysts, which could establish strong interfacial electronic coupling to greatly facilitate the separation/migration of photogenerated electron-hole pairs and optimize the HER performance of the reactive sites on NiPS 3 UNSs. In detail, the as-prepared 20.0 ml of NiPS 3 UNSs ethanol solution was merged with 50 mg of four different semiconductor photocatalysts, respectively, which include metal oxide (TiO 2 ), metal sulfides (CdS and In 2 ZnS 4 ) and metal-free nitride (C 3 N 4 ). The resulting hybrid photocatalysts were denoted, respectively, as NiPS 3 /TiO 2 , NiPS 3 /CdS, NiPS 3 /In 2 ZnS 4 and NiPS 3 /C 3 N 4 . The photocatalytic H 2 -production rates of all the hybrid photocatalysts exhibit an apparent improvement in contrast to the photocatalysts without NiPS 3 (Fig. 1i ). Among them, NiPS 3 /CdS shows the highest photocatalytic H 2 -production rate (13,600 μmol h −1 g −1 ), surpassing that of bare CdS (816 μmol h −1 g −1 ) by ~1667%. These results show that NiPS 3 UNSs could serve as a versatile and highly active platform to enhance the photocatalytic H 2 -production rates on various kinds of photocatalysts. Since the NiPS 3 /CdS system presents the highest photocatalytic H 2 -production rate (13,600 μmol h −1 g −1 ) and largest enhancement factor (~1667%), a range of experiments and theoretical computations were performed to investigate this representative NiPS 3 /CdS system. Phase structure, morphology and strong electronic interaction of NiPS 3 /CdS heterojunction First, pure CdS NPs synthesized via a hydrothermal approach were studied using HAADF-STEM, elemental mapping, EDX spectroscopy and Raman spectroscopy. The HAADF-STEM image of CdS NPs (Supplementary Fig. 11a ) shows the sizes of ~11–36 nm for CdS NPs. The high-resolution HAADF-STEM image of CdS NPs (Supplementary Fig. 11b ) presents the two lattice spacing values of 0.34 and 0.34 nm, together with an angle of 70.5°, attributed, respectively, to the (111) and (11−1) facets of cubic CdS. Moreover, the HAADF-STEM image (Supplementary Fig. 11c ) and corresponding elemental mapping images (Supplementary Fig. 11d, e ) of CdS NPs further indicate the successful preparation of CdS NPs. The EDX spectrum of CdS NPs (Supplementary Fig. 11f ) indicates the presence of Cd and S elements in agreement with the above results. The Raman spectrum of CdS NPs in Supplementary Fig. 12 confirms the presence of typical 1LO, 2LO and 3LO peaks for CdS in agreement with the previous work [66] . Then, different volumes of NiPS 3 UNSs ethanol solution (5.0, 10.0, 20.0 and 30.0 ml) were, respectively, added to a mortar to couple with 50 mg of the as-prepared CdS NPs via mechanical grinding at room temperature. The resulting photocatalysts were, respectively, labelled as 5.0N, 10.0N, 20.0N and 30.0N. Pure CdS NPs were denoted as 0.0N. First, the phase structures of all the as-prepared samples were revealed by X-ray diffraction (XRD). The XRD patterns of 0.0N, 5.0N, 10.0N, 20.0N and 30.0N are displayed in Supplementary Fig. 13 . All the samples exhibit a Hawleyite cubic-phase structured CdS (JCPDS #10-0454). No apparent alteration of the intensities and positions of diffraction peaks are observed for 5.0N, 10.0N, 20.0N and 30.0N, in contrast with those of 0.0N (Supplementary Fig. 13 ). These results suggest that the physical mixing of CdS NPs with NiPS 3 UNSs at room temperature does not impact the original crystal structure of CdS NPs. Moreover, the absence of NiPS 3 diffraction peak in 5.0N, 10.0N, 20.0N and 30.0N arises from the low content and homogeneous dispersion of NiPS 3 UNSs. Then, the morphology, microstructure and compositions of 20.0N were explored. 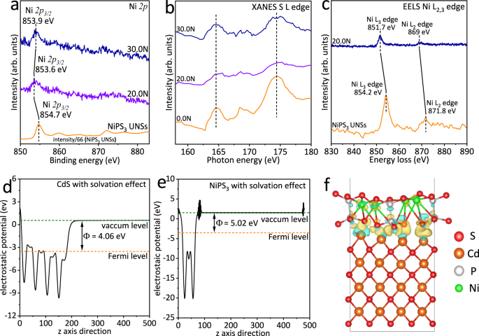The TEM image of 20.0N is shown in Fig. 2a . CdS NPs with sizes of ~15–39 nm are uniformly dispersed onto the surface of NiPS 3 UNSs. Fig. 3: Strong electronic interaction in NiPS3/CdS system. aHigh-resolution XPS spectra of Ni2pfor NiPS3UNSs, 20.0N and 30.0N.bSynchrotron-based XANES S L edge of 0.0N, 20.0N and 30.0N.cEELS spectra of Ni L2,3edge for NiPS3UNSs and 20.0N. Average potential profiles along thezaxis direction ofdCdS (200) crystal facet andeNiPS3(002) crystal facet.fThe differential charge density map of NiPS3/CdS system. The golden and cyan iso-surfaces indicate the area of net-electron accumulation and deficit, respectively. The work functions and differential charge density map were calculated considering the solvation effect in 17 vol% triethanolamine aqueous solution. The HRTEM image in Fig. 2b further shows two lattice spacing values of 0.30 and 0.34 nm, together with an angle of 125.3°. These two crystal planes are ascribed to the (00−2) and (111) facets of cubic CdS, respectively. Besides, the other two lattice spacing values of 0.29 and 0.29 nm, and an angle of 117.9° are also displayed in Fig. 2b . These two crystal planes are, respectively, assigned to the (130) and (1−30) planes of monoclinic NiPS 3 . 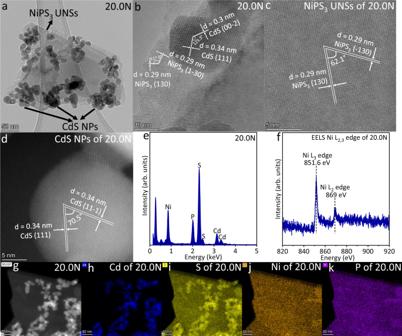The above results further confirm the successful loading of CdS NPs onto NiPS 3 UNSs. The atomic-resolution HAADF-STEM image of NiPS 3 UNSs in 20.0N (Fig. 2c ) displays two lattice spacing values of 0.29 and 0.29 nm, accompanied by an angle of 62.1°. These two facets are ascribed to the (130) and (−130) planes of monoclinic NiPS 3 UNSs, respectively. Fig. 2: Morphology, microstructure, and chemical compositions of 20.0N. aTEM image andbHRTEM image of 20.0N. Atomic-resolution HAADF-STEM images ofcNiPS3UNSs anddCdS NPs in 20.0N.eEDX spectrum of 20.0N.fEELS spectrum of Ni L2,3edge for 20.0N.gHAADF-STEM image of 20.0N and the corresponding elemental mapping images ofhCd,iS,jNi andkP elements in 20.0N. Figure 2d exhibits the atomic-resolution HAADF-STEM image of CdS NPs in 20.0N. Two lattice spacing values of 0.34 and 0.34 nm, as well as an angle of 70.5° are observed in Fig. 2d , corresponding to (111) and (11−1) facets of cubic CdS. The EDX spectrum of 20.0N (Fig. 2e ) suggests the existence of Cd, S, Ni and P elements, in accordance with the above results. The electron energy loss spectroscopy (EELS) pattern of Ni L 2,3 edges for 20.0N (Fig. 2f ) shows that the Ni L 2 edge and Ni L 3 edge are located at 869 and 851.6 eV, respectively. Moreover, the HAADF-STEM image of 20.0N (Fig. 2g ) further shows that many CdS NPs are loaded onto the surface of NiPS 3 UNSs. The much brighter CdS NPs than NiPS 3 NSs in Fig. 2g arises from the much larger atomic number of Cd (Z = 48) compared with those of Ni (Z = 28), P (Z = 15) and S (Z = 16). The corresponding elemental mapping images of Cd (Fig. 2h ), S (Fig. 2i ), Ni (Fig. 2j ) and P (Fig. 2k ) are in accordance with the HAADF-STEM image of 20.0N (Fig. 2g ). All the above results support the successful merging of CdS NPs with NiPS 3 UNSs in 20.0N. XPS analysis, which can reveal the surface element status, was adopted to detect the interfacial electronic interaction between CdS NPs and NiPS 3 UNSs. As shown in Fig. 3a , the Ni 2p 3/2 peaks of 20.0N and 30.0N exhibit the obvious left shift toward the low binding energy direction, in contrast with that of NiPS 3 UNSs. These results disclose the electron transfer from CdS NPs to NiPS 3 UNSs after combining CdS NPs and NiPS 3 UNSs in 20.0N and 30.0N. Notably, in comparison with the Ni 2p 3/2 peak of NiPS 3 UNSs, the Ni 2p 3/2 peak of 20.0N shows a left shift of 1.1 eV; while the Ni 2p 3/2 peak of 30.0N exhibit a smaller left shift of 0.8 eV (Fig. 3a ). This is attributed to the higher amount of NiPS 3 UNSs in 30.0N than that in 20.0N. Moreover, compared to the Cd 3d and S 2p peaks of 0.0N (CdS NPs) in Supplementary Fig. 14a, b , no obvious shift of Cd 3d and S 2p peaks is observed in 20.0N and 30.0N, which is due to the following two reasons: (1) the weight amount of CdS NPs is much larger than that of NiPS 3 UNSs in 20.0N or 30.0N. 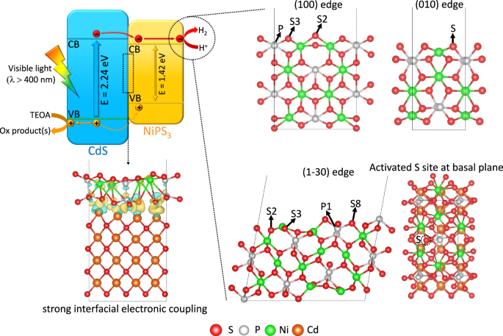Fig. 7: Schematic illustration of photocatalytic H2-production mechanism in NiPS3/CdS system. The visible-light excitation (λ> 400 nm), separation/migration of photogenerated electrons and holes, and the surface catalytic reactions of NiPS3/CdS system are shown in the figure. This is corroborated by the inductively coupled plasma atomic emission spectroscopy (ICP-AES) test, displaying the weight amount of NiPS 3 UNSs (3.603 wt%) in 20.0N (Supplementary Table 7 ); (2) some CdS NPs tend to aggregate rather than contact with NiPS 3 UNSs in 20.0N and 30.0N. In addition, the synchrotron-based X-ray absorption near edge structure (XANES) S L edges of 20.0N and 30.0N exhibit no obvious shift in contrast with that of 0.0N (Fig. 3b ), which agrees with the aforementioned XPS results. Furthermore, the EELS Ni L 2,3 edges for 20.0N show the apparent shift (2.5 or 2.8 eV) toward the low energy direction, in contrast with those of NiPS 3 UNSs (Fig. 3c ). This obvious shift is because the EELS Ni L 2,3 edge spectrum was acquired in the selected region, where CdS NPs contact with NiPS 3 UNSs. Hence, the EELS spectra (Fig. 3c ) also corroborate the electron migration from CdS NPs to NiPS 3 UNSs. Moreover, the Mott-Schottky plots in Supplementary Figs. 15 and 9a show that the flat band potentials of CdS NPs and NiPS 3 UNSs are -0.89 and -0.58 V vs. Ag/AgCl electrode, corresponding to the −0.26 and 0.05 V vs. SHE. Thus, the E F value for CdS NPs is more negative than that of NiPS 3 UNSs. As a result, electrons would migrate from CdS NPs to NiPS 3 UNSs via the interface in 20.0N. Furthermore, as shown in Fig. 3d, e , the work functions (Φ) of CdS (200) crystal facet and NiPS 3 (002) crystal facet are, respectively, calculated to be 4.06 and 5.02 eV. These results also support the electron extraction from CdS to NiPS 3 at the interface after combining CdS and NiPS 3 . Besides, the differential charge density map at the interface of CdS and NiPS 3 (Fig. 3f ) also suggests the interfacial electron transport from CdS to NiPS 3 after coupling them. The Bader charge transferred from CdS to NiPS 3 is │1.34│e, also in support of the electron migration from CdS to NiPS 3 . Moreover, the spin-up and spin-down electronic band structures and density of states (DOS) for CdS and NiPS 3 were calculated, respectively. As displayed in Supplementary Fig. 16a, b , both the conduction band minimum (CBM) and valence band maximum (VBM) of CdS are located at the X point of the Brillouin zone with the direct band gap transition. The calculated direct (ΔE) band gap between CBM and VBM of CdS is 1.90 eV, which is close to the experimental value [13] . The spin-up and spin-down DOS of CdS (Supplementary Fig. 16c ) also show the same band gap (Δ E = 1.90 eV), in accordance with the calculated band structures (Supplementary Fig. 16a, b ). Moreover, NiPS 3 shows the spin-polarized electronic band structures with a direct spin-up band gap of 1.75 eV (Supplementary Fig. 16d ) and indirect spin-down band gap of 1.83 eV (Supplementary Fig. 16e ), in agreement with the calculated and experimental results [52] , [57] . And the spin-up and spin-down DOS of NiPS 3 (Supplementary Fig. 16f ) display an identical band gap (Δ E = 1.75 eV), in agreement with the calculated band structures (Supplementary Fig. 16d, e ). Fig. 2: Morphology, microstructure, and chemical compositions of 20.0N. a TEM image and b HRTEM image of 20.0N. Atomic-resolution HAADF-STEM images of c NiPS 3 UNSs and d CdS NPs in 20.0N. e EDX spectrum of 20.0N. f EELS spectrum of Ni L 2,3 edge for 20.0N. g HAADF-STEM image of 20.0N and the corresponding elemental mapping images of h Cd, i S, j Ni and k P elements in 20.0N. Full size image Fig. 3: Strong electronic interaction in NiPS 3 /CdS system. a High-resolution XPS spectra of Ni 2p for NiPS 3 UNSs, 20.0N and 30.0N. b Synchrotron-based XANES S L edge of 0.0N, 20.0N and 30.0N. c EELS spectra of Ni L 2,3 edge for NiPS 3 UNSs and 20.0N. Average potential profiles along the z axis direction of d CdS (200) crystal facet and e NiPS 3 (002) crystal facet. f The differential charge density map of NiPS 3 /CdS system. The golden and cyan iso-surfaces indicate the area of net-electron accumulation and deficit, respectively. The work functions and differential charge density map were calculated considering the solvation effect in 17 vol% triethanolamine aqueous solution. Full size image The presence of strong electronic interaction at the interface between CdS and NiPS 3 is confirmed by both the above experimental results and theoretical calculations. To further corroborate that NiPS 3 UNSs can establish a strong electronic coupling between various semiconductor photocatalysts, we have conducted a range of high-resolution XPS studies for NiPS 3 /TiO 2 (Supplementary Fig. 17a–d ), NiPS 3 /In 2 ZnS 4 (Supplementary Fig. 17e–h ) and NiPS 3 /C 3 N 4 (Supplementary Fig. 17i–l ). All the results confirm the electrons migration from TiO 2 , In 2 ZnS 4 or C 3 N 4 to NiPS 3 UNSs, as evidenced by the pronounced shift of high-resolution XPS peaks (Supplementary Fig. 17a–l ). Excellent photocatalytic performance of NiPS 3 /CdS heterojunction The photocatalytic H 2 -production rates of all the as-synthesized samples were examined in ~17 vol% triethanolamine aqueous solution with visible-light illumination ( λ > 400 nm). 0.0N (pure CdS NPs) presents a low photocatalytic H 2 -production rate of 816 μmol h −1 g −1 (Fig. 4a ) owing to the fast recombination of photoinduced electron-hole pairs and insufficient active sites on the surface. After combining CdS NPs with NiPS 3 UNSs, 5.0N exhibits an obviously-increased photocatalytic H 2 -production rate (2946 μmol h −1 g −1 ). Further increase in the NiPS 3 UNSs amount results in an even larger photocatalytic H 2 -production rate of 5208 μmol h −1 g −1 on 10.0N. Remarkably, 20.0N exhibits the largest photocatalytic H 2 -production rate (13,600 μmol h −1 g −1 ). This excellent activity is ranked among the most efficient noble-metal-free CdS-based photocatalysts (Supplementary Table 8 ). Besides, this activity is also higher than the other MPC x -based photocatalysts (Supplementary Table 9 ) [50] , [51] , [52] , [53] , [54] , [55] , such as Eosin Y-sensitized NiPS 3 sheets (2600 μmol h −1 g −1 ) [53] , NiPS 3 nanosheets covered carbon fibre (74.67 μmol h −1 g −1 ) [52] , FePS 3 nanosheets (402.4 μmol h −1 g −1 ) [55] and MnPSe 3 nanosheets covered carbon fibre (43.5 μmol h −1 g −1 ) [50] . These results also support that NiPS 3 is better to be combined with another photocatalyst rather than being used alone for achieving a further raise in photocatalytic H 2 -production activity. Additionally, 20.0N shows an apparent quantum yield (AQY) of 20.2% at 420 nm, ranking as one of the most active noble-metal-free CdS-based photocatalysts (Supplementary Table 8 ). Nevertheless, we have also noticed that some works reported higher photocatalytic H 2 -production rates and AQYs as displayed in Supplementary Table 8 . For instance, MoS 2 /CdS heterostructure shows a photocatalytic H 2 -production rate of 49,800 μmol h −1 g −1 in lactic acid aqueous solution under visible-light illumination [14] . Besides, this heterostructure also displays an AQY of 41.37% at 420 nm. In another work, WO 3 /CdS/WS 2 direct Z -scheme heterojunction exhibits a photocatalytic H 2 -production rate of 14,340 μmol h −1 g −1 in lactic acid aqueous solution with visible light irradiation [36] . And an AQY of 22.96% at 435 nm was also achieved on this heterojunction. However, the above rates and AQYs were acquired in the photocatalytic test systems with different reaction conditions, such as weight of catalyst, pH value of reaction solution and type/concentration of sacrificial reagent. Apart from the intrinsic activities of photocatalysts, these factors can also affect the above rates and AQYs [33] , [34] , [35] . On the other hand, the Mo and W elements in MoS 2 and WS 2 , respectively, possess a much lower abundance (1.20 and 1.25 ppm for Mo and W, respectively) than that of Ni element (84.00 ppm) in Earth’s crust [67] . Thus, the NiPS 3 UNSs developed in our work are a more cost-effective platform for advancing photocatalytic H 2 production, compared with MoS 2 or WS 2 . Notably, a further increase in the NiPS 3 UNSs amount results in a decrease in the photocatalytic H 2 -production rate to 10,044 μmol h −1 g −1 on 30.0N, possibly due to the excessive NiPS 3 UNSs partially blocking light harvesting and covering surface active sites. We also tested the photocatalytic H 2 -production rate of pure NiPS 3 UNSs. However, no H 2 production was observed on pure NiPS 3 UNSs under the same reaction conditions, probably due to the weak oxidation abilities of photogenerated holes in the VB of NiPS 3 UNSs (Supplementary Fig. 10 ). Thus, the photogenerated holes cannot oxidize the sacrificial electron donor, triethanolamine, leading to the fast recombination of photo-generated electron-hole pairs. Fig. 4: Photocatalytic H 2 -production activities and charge carrier kinetics of NiPS 3 /CdS system. a Photocatalytic H 2 -production rates of 0.0N, 5.0N, 10.0N, 20.0N, 30.0N and NiPS 3 UNSs in ~17.0 vol% triethanolamine aqueous solution using visible-light illumination ( λ > 400 nm). b Steady-state and c transient-state PL spectra of 0.0N and 20.0N. c Inset shows the fitting charge lifetimes for 0.0N and 20.0N. 2D pseudocolor TA spectra of d 0.0N and e 20.0N in ethanol solution after the excitation with a 400 nm laser pulse. The TA spectra of f 0.0N and g 20.0N at different pump-probe delay time. h Normalized decay kinetics and fitting lines for 0.0N and 20.0N taken through the GSB peaks at ~516 and ~514 nm, respectively. i Normalized decay kinetics and fitting lines for 0.0N and 20.0N taken through the ESA peaks at ~480 and ~474 nm, respectively. Full size image The stability of 20.0N was also tested for four cycles. The H 2 -production amount in the fourth cycle accounts for 49.17% of that in the first hour (Supplementary Fig. 18 ). To find the reason for the reduced activity, we have conducted the XRD, TEM, EDX and atomic-resolution HAADF-STEM characterizations for 20.0N after the 4-h reaction (20.0N-A). As shown in Supplementary Fig. 19 , there is a slight reduction in the peak intensities of the XRD peaks for 20.0N-A compared to those of 20.0N, suggesting the weakened crystallinity of CdS NPs after the reaction. However, the TEM image (Supplementary Fig. 20a ) and EDX spectrum (Supplementary Fig. 20b ) of 20.0N-A show that no obvious alteration in the morphology and chemical compositions is found for 20.0N-A in comparison to those of 20.0N (Fig. 2a, e ). Thus, the atomic-resolution HAADF-STEM images of 20.0N-A were explored. We found that the amorphous region appears on the surface of CdS NPs (Supplementary Fig. 20c ) and at the edge of NiPS 3 UNSs (Supplementary Fig. 20d ). It seems that the generation of an amorphous region on the surface of CdS NPs (Supplementary Fig. 20c ) led to the reduced crystallinity of CdS NPs in 20.0N-A (Supplementary Fig. 19 ). Notably, since abundant H 2 -evolution active sites exist at the edges of NiPS 3 UNSs, the structure destruction at the edges of NiPS 3 UNSs resulted in the reduced H 2 -production activity of 20.0N-A (Supplementary Fig. 18 ). To further explore the stability of 20.0N, we have tested its stability in 0.35 M Na 2 S and 0.25 M Na 2 SO 3 aqueous solution, which is usually applied as the sacrificial electron donor to inhibit the self-corrosion of metal sulfide photocatalysts. However, a similar reduction of activity in the second to the fourth hour is also observed in 0.35 M Na 2 S and 0.25 M Na 2 SO 3 aqueous solution (Supplementary Fig. 21 ). And we have acquired the TEM image, EDX spectrum and atomic-resolution HAADF-STEM images of 20.0N after the four-hour reaction in Na 2 S and Na 2 SO 3 aqueous solution (20.0N-A-S) as shown in Supplementary Fig. 22a–d . No apparent difference is observed in the morphology (Supplementary Fig. 22a ) and chemical compositions (Supplementary Fig. 22b ) of 20.0N-A-S, in comparison to those of 20.0N (Fig. 2a, e ). However, the atomic-resolution HAADF-STEM images of 20.0N-A-S reveal the existence of an amorphous region on the surface of CdS NPs (Supplementary Fig. 22c ) and at the edge of NiPS 3 UNSs (Supplementary Fig. 22d ), respectively. These are attributed to the photo-corrosion caused by the photogenerated holes in 20.0N, thus indicating that Na 2 S/Na 2 SO 3 , unfortunately, cannot effectively impede the photo-corrosion on CdS NPs and NiPS 3 UNSs in this work. Kinetics and thermodynamics of photogenerated electrons/holes in NiPS 3 /CdS heterojunction The origin of the excellent photocatalytic performance on 20.0N was investigated by both the advanced characterizations and theoretical computations. Since the interfacial charge separation/migration serves a pivotal role in the whole photocatalysis process, the dissociation and transport of photogenerated electrons/holes were investigated using a range of advanced characterizations, including steady-state and transient-state photoluminescence (PL) spectroscopy, ultrafast transient absorption spectroscopy (TAS), steady-state and transient-state surface photovoltage (SPV) spectroscopy, light-irradiated contact potential difference (CPD) test, in situ XPS, and transient photocurrent (TPC) density measurements. To study the charge carrier separation and migration, we need to determine the heterojunction type of NiPS 3 /CdS system first. As shown in Supplementary Fig. 23a , the VB edge of 0.0N (CdS NPs) is 1.72 V vs. the E F of 0.0N. Since the E F of 0.0N is decided to be −0.26 V vs. SHE (Supplementary Fig. 15 ), the VB edge of 0.0N (CdS NPs) is 1.46 V vs. SHE. Thus, the CB edge of 0.0N (CdS NPs) is −0.78 V vs. SHE, based on the band gap value ( E = 2.24 eV; Supplementary Fig. 23b ). Therefore, as shown in Supplementary Fig. 24, a type I (straddling type) heterojunction is formed in the NiPS 3 /CdS system. However, type I heterojunction is usually not regarded as an effective heterostructure, since both photogenerated electrons and holes would migrate to the same semiconductor with a smaller band gap width. This would lead not only to the decreased redox abilities of electrons and holes but also to the inefficient dissociation of electrons and holes. But NiPS 3 /CdS system has achieved a very high photocatalytic H 2 -production rate (Fig. 4a ). So, various state-of-art characterizations were performed to understand the kinetics and thermodynamics of photogenerated charge carriers in NiPS 3 /CdS system (20.0N). Both the steady-state and transient-state PL spectroscopy measurements were performed to study the radiative recombination of photo-generated electrons/holes in 20.0N. The steady-state PL spectra of 0.0N and 20.0N are displayed in Fig. 4b . 0.0N show a PL peak at ~563 nm, due to the radiative band-to-band recombination of photogenerated electrons and holes. In comparison, 20.0N exhibits a depressed PL peak, indicating that the radiative band-to-band recombination in 20.0N is suppressed compared to that of 0.0N. Furthermore, the transient-state PL spectra of 0.0N and 20.0N are presented in Fig. 4c . The charge carrier lifetimes were calculated for 0.0N and 20.0N via bi-exponential fitting of the transient-state PL spectra in Fig. 4c . The as-acquired short ( τ 1 ), long ( τ 2 ) and intensity-averaged ( τ ave ) lifetimes for 0.0N and 20.0N are displayed in Fig. 4c inset. The short lifetime ( τ 1 ) is mainly caused by the radiative pathways; while the long lifetime ( τ 2 ) is related to the non-radiative behaviour [11] . As shown in Fig. 4c inset, 20.0N exhibits a longer τ 1 (0.20 ns) for a majority of charge carriers (97.85%), a prolonged τ 2 (6.67 ns) for a very small content of charge carriers (2.15%) and an elongated τ ave (0.34 ns), in comparison to 0.0N ( τ 1 = 0.18 ns; τ 2 = 4.74 ns; τ ave = 0.30 ns). As a result, the transient-state PL spectra and the corresponding lifetime fitting results together confirm that the charge carrier separation/transport in 20.0N is promoted in contrast to that in 0.0N. Ultrafast TAS is a powerful technique for understanding behaviour of light-induced electrons and holes in photocatalysts. Hence, we used TAS to explore the charge carrier dynamics of 0.0N and 20.0N dispersed in ethanol after a 400 nm laser pulse with an energy of 0.1 μJ. As displayed in Fig. 4d, e , both the TA spectra of 0.0N and 20.0N show distinct negative and positive absorption bands, which are assigned, respectively, to the ground-state bleaching (GSB) and excited-state absorption (ESA) signals. Moreover, the ultrafast TA spectra of 0.0N and 20.0N at different pump-probe delay times are, respectively, displayed in Fig. 4f, g . The redshifts of the GSB peaks over time can be observed in both Fig. 4f, g . This is because CdS NPs in 0.0N and 20.0N possess a broad size distribution, in which the smaller CdS NPs have the larger band gaps and the faster exciton annihilation [68] . To further explore the detailed dynamic behaviours of photogenerated charge carriers, the GSB and ESA decay kinetics of both 0.0N and 20.0N are shown in Fig. 4h, i , respectively. All the fitting results are presented in Supplementary Table 10 accordingly. The suppressed GSB (Fig. 4h ) and ESA (Fig. 4i ) kinetic decays in the probing timescale are visible in comparison to that of 0.0N. These findings are further supported by the three-exponential fitting results of TA spectra for 0.0N and 20.0N (Supplementary Table 10 ). Since the three-exponential fitting results of 0.0N and 20.0N samples (Supplementary Table 10 ) indicate the existence of long-lived lifetime ( τ > 3 ns), we have also collected the long-time TA spectra of 0.0N and 20.0N (up to 7.73 ns) and the results are shown in Supplementary Fig. 25a, b , respectively. The obvious negative absorption bands can be observed in both Supplementary Fig. 25a, b , ascribed to the GSB signals. Supplementary Fig. 25c, d show the ultrafast TA spectra of 0.0N and 20.0N at different pump–probe delay times, respectively. The GSB decay kinetics of 0.0N and 20.0N in the range of 0–7.73 ns and the corresponding fitting results are displayed in Supplementary Fig. 25e and Supplementary Table 11 , respectively. Both the impeded GSB decay kinetics (Supplementary Fig. 25e ) and elongated fitting lifetimes (Supplementary Table 11 ) of 20.0N compared to those of 0.0N are in accordance with the above results. Hence, the TAS results also corroborate that the coupling of NiPS 3 UNSs with CdS NPs efficiently impedes the charge carrier recombination in 20.0N. Since photocatalysis mainly involves the charge carriers at the surface/interface of photocatalysts, the behaviours of charge carriers at the surface/interface of photocatalysts were explored using a range of state-of-art techniques, such as steady-state and transient-state SPV spectroscopy, light-irradiated CPD test, and in situ XPS test. As can be seen in the transient-state SPV spectrum of 0.0N (Fig. 5a ), after the excitation with a 355-nm pulse laser, a negative SPV signal is observed for 0.0N. This result indicates that compared to photo-generated holes, more photo-generated electrons migrate from the bulk to the surface of 0.0N (CdS NPs). In contrast, 20.0N exhibits a positive SPV signal in Fig. 5a . This result suggests that the loading of CdS NPs onto NiPS 3 UNSs apparently boosts the migration of photo-generated holes from the bulk to the surface. This is attributed to the establishment of type I heterojunction between CdS NPs and NiPS 3 UNSs, which promotes both the photogenerated electrons and holes in the CB and VB of CdS NPs to the CB and VB of NiPS 3 UNSs, respectively (Supplementary Fig. 24 ). Notably, as displayed in Supplementary Fig. 24 , the potential difference (0.60 V) between the VB edges of CdS NPs and NiPS 3 UNSs is much larger than the potential difference (0.22 V) between the CB edges of CdS NPs and NiPS 3 UNSs. From the viewpoint of thermodynamics, compared with the photogenerated electrons in CdS NPs, the photogenerated holes in CdS NPs would migrate more efficiently to NiPS 3 UNSs in 20.0N. Thus, with light excitation, more photogenerated holes would accumulate on the surface/interface of CdS NPs and NiPS 3 UNSs in 20.0N, resulting in a positive SPV signal in Fig. 5a . Furthermore, Fig. 5a shows that for 20.0N the absolute value of the SPV signal is reduced as compared with that of 0.0N. This is because both photogenerated electrons and holes are promoted to migrate from CdS NPs to NiPS 3 UNSs, leading to the accumulation of both photogenerated electrons and holes on the surface/interface. As a result, for 20.0N the net value of the positive SPV signal is reduced in contrast with that of 0.0N. This is further supported by the steady-state SPV spectra of 0.0N and 20.0N (Fig. 5b ) showing that for 20.0N the absolute value of the SPV signal is smaller than that of 0.0N. Moreover, Fig. 5c shows that the CPD value of 0.0N (CdS NPs) is rapidly decreased from 550 mV in the dark to 250 mV under light irradiation. This result suggests that under light excitation more photogenerated electrons than holes migrate from the bulk to the surface of CdS NPs, resulting in the upward band bending and improvement of E F . This phenomenon is in accordance with the negative value of the transient-state SPV signal for 0.0N (Fig. 5a ). Fig. 5: Charge carrier kinetics in NiPS 3 /CdS system. a Transient-state and b steady-state SPV spectra of 0.0N and 20.0N. c CPD test of 0.0N in the dark and under light irradiation. High-resolution XPS spectra of d Ni 2p , e P 2p and f S 2p of NiPS 3 UNSs with the light on and off, respectively. High-resolution XPS spectra of g Ni 2p , h Cd 3d and i S 2p of 20.0N with the light on and off, respectively. Full size image Furthermore, the in situ XPS tests were also conducted to reveal the dissociation and migration of photo-generated electrons and holes on/near the surface of photocatalysts. As shown in Fig. 5d–f , the Ni 2p , P 2p and S 2p peaks for NiPS 3 UNSs shift to the high binding energy direction by 0.2–0.4 eV under light irradiation as compared to those in the dark. These results disclose that more photogenerated holes than electrons transfer from the bulk to the surface of NiPS 3 UNSs under light illumination. Further studies show that the Ni 2p (Fig. 5g ), Cd 3d (Fig. 5h ) and S 2p (Fig. 5i ) peaks observed for 20.0N move toward the high binding energy, suggesting that for this system more photogenerated holes than electrons migrate to the surface of both CdS NPs and NiPS 3 UNSs after light excitation. These results are in accordance with the positive transient-state SPV signal of 20.0N (Fig. 5a ). However, it should be noted that the steady-state/transient-state SPV spectroscopy tests, in situ XPS tests and light-irradiated CPD test were all performed using dry powder-form of the photocatalysts, in the absence of sacrificial electron donor (triethanolamine). But in realistic photocatalytic H 2 -production tests, 0.0N or 20.0N were first dispersed in triethanolamine aqueous solution under constant stirring. Hence, these photogenerated holes migrating to the surface of CdS NPs would be rapidly captured by the sacrificial electron donor, triethanolamine, leaving the photogenerated electrons for H 2 evolution. Furthermore, the transient photocurrent (TPC) density measurement (Supplementary Fig. 26 ) displays that 20.0N electrode possesses a larger anodic current density than that of 0.0N electrode. This is ascribed to the two following reasons: (1) for 20.0N having NiPS 3 UNSs, more photoinduced holes are transported to the surface and interface, favouring the oxidation reaction occurring at the electrode/electrolyte interface; (2) for 20.0N the promoted electron–hole separation/transfer leads to more photoinduced electrons transferred to the counter electrode for reduction reaction. Surface catalytic redox reactions and light absorption/excitation of NiPS 3 /CdS heterojunction Apart from charge carrier separation/migration, the surface catalytic redox reactions and light absorption/excitation are the other two major factors affecting the whole photocatalysis process. For the surface catalytic redox reactions, we focus on the reduction reaction or HER on NiPS 3 /CdS (20.0N). Figure 6a presents the linear sweep voltammetry (LSV) curves for 0.0N, 20.0N, NiPS 3 UNSs and 20 wt% Pt/C in 0.1 M KOH aqueous solution. Pure NiPS 3 UNSs exhibit excellent HER activity (Fig. 6a ), although the HER activity of NiPS 3 UNSs is inferior to that of 20 wt% Pt/C. 20.0N presents a superior HER activity in contrast to that of 0.0N, due to the presence of NiPS 3 UNSs with abundant atomic-level edge P/S active sites. Besides, the HER electrochemical stability tests for NiPS 3 UNSs, NiPS 3 /TiO 2 , 20.0N, NiPS 3 /In 2 ZnS 4 and NiPS 3 /C 3 N 4 at the potential of −0.6 V vs. RHE are displayed in Supplementary Fig. 27a–e , respectively. The above results support that NiPS 3 UNSs and all the composites possess excellent HER stability in 0.1 M KOH aqueous solution. This further indicates that the NiPS 3 UNSs will not be corroded in the reduction environment in an alkaline solution. And the results also suggest the photo-generated hole is the reason causing the deactivation of NiPS 3 UNSs active sites. Additionally, the DFT-based computations reveal that the combination of NiPS 3 with CdS leads to the greatly-reduced Δ G H* values on P and S sites at the basal plane of NiPS 3 monolayer in NiPS 3 /CdS system (Fig. 6b–d and Supplementary Table 12 ), in comparison to those of pure NiPS 3 monolayer (Supplementary Fig. 1a–c and Supplementary Table 2 ). Especially, the inactive S site on the basal plane of NiPS 3 monolayer becomes much more active in NiPS 3 /CdS system for HER following the Volmer-Heyrovsky pathway (Supplementary Tables 2 and 12 ). In contrast, the ΔG H* values on Ni site at the basal plane of NiPS 3 monolayer in NiPS 3 /CdS are obviously increased for the first Volmer step (Supplementary Table 12 ), compared to the Ni site at the basal plane of NiPS 3 monolayer alone (Supplementary Table 2 ). This result suggests the reduced HER activity of Ni site after the combination of NiPS 3 and CdS. Overall, the strong electronic combination of NiPS 3 with CdS leads to the activated S site of NiPS 3 monolayer in NiPS 3 /CdS system. For the surface catalytic oxidation reaction, since more photogenerated holes migrate to the surface of 20.0N after coupling CdS and NiPS 3 , the oxidation of electron donor, triethanolamine, to the oxidation product(s) is facilitated. Moreover, the N 2 sorption isotherm measured for 20.0N shifts downs compared with that of 0.0N (Supplementary Fig. 28 ). Consequently, the Brunauer–Emmett–Teller (BET) surface area and pore volume evaluated for 20.0N are also slightly lower than those obtained for 0.0N (Supplementary Table 7 ). This is due to the mild aggregation of CdS NPs in 20.0N after evaporating ethanol in the physical mixing process. These results also indicate that the surface area does not have a significant impact on the photocatalytic activity of NiPS 3 /CdS system. Fig. 6: Surface catalytic reactions and light absorption of NiPS 3 /CdS system. a Electrochemical HER activities in 0.1 M KOH aqueous solution for 0.0N, 20.0N, NiPS 3 UNSs and 20 wt% Pt/C. b top-view atomic structure of NiPS 3 /CdS showing the Ni, P and S basal sites. c The calculated free energy diagrams of HER following the Volmer-Heyrovsky pathway on the Ni, P and S sites of NiPS 3 basal plane in NiPS 3 /CdS system. d The calculated free energy diagrams of HER following the Volmer-Tafel pathway on the Ni, P and S sites of NiPS 3 basal plane in NiPS 3 /CdS system. e UV-Vis diffuse reflectance spectra of 0.0N, 5.0N, 10.0N, 20.0N and 30.0N. f Photocatalytic H 2 -production rates measured for 20.0N in ~17.0 vol% triethanolamine aqueous solution with xenon light irradiation ( λ > 400 nm) and 630-nm LED, respectively. All the Gibbs free energy calculations were conducted considering the solvation effect in 17 vol% triethanolamine aqueous solution. Full size image Since NiPS 3 UNSs possess a small band gap of 1.42 eV with a wide light absorption spectrum (up to 873 nm), intensified visible-light absorption is observed for 5.0N, 10.0N, 20.0N and 30.0N (Fig. 6e ). The visible-light absorption is gradually improved with an increasing amount of NiPS 3 UNSs, i.e, from 5.0N, 10.0N, 20.0N to 30.0N (Fig. 6e ). To study whether the increased visible-light absorption of 20.0N (Fig. 6e ) contributed to the high H 2 -production rate (Fig. 4a ), we tested the photocatalytic H 2 -production rate of 20.0N under 630-nm light emitting diode (LED) illumination. However, 20.0N exhibits a negligible photocatalytic H 2 production under 630-nm LED light irradiation (Fig. 6f ). This is because the photons of 630-nm LED light ( hν = 1.97 eV) can only excite NiPS 3 UNSs rather than CdS NPs. However, the weak photogenerated holes in the VB of NiPS 3 UNSs (Supplementary Fig. 10 ) cannot oxidize the electron donor, triethanolamine. Thus, the photogenerated electrons and holes rapidly recombine with each other, leading to negligible photocatalytic H 2 production on pure NiPS 3 UNSs. This also suggests that the strengthened absorption observed for NiPS 3 UNSs (Fig. 6e ) does not contribute to the improved photocatalytic activity. Photocatalytic mechanism for NiPS 3 /CdS heterojunction Based on the aforementioned experiments and calculations, a photocatalytic mechanism is proposed for the NiPS 3 /CdS heterojunction (Fig. 7 ). First, under visible-light irradiation ( λ > 400 nm), both CdS NPs and NiPS 3 UNSs are excited and photoinduced electrons and holes are, respectively, generated on the CB and VB. Due to the formation of type I heterojunction (straddling type) between CdS NPs and NiPS 3 UNSs, together with the strong interfacial electronic coupling between CdS NPs and NiPS 3 UNSs (Fig. 7 ), the photoinduced electrons and holes should, respectively, migrate from the CB and VB of CdS NPs to those of NiPS 3 UNSs. However, in the existence of a sacrificial electron donor, triethanolamine, most of the photogenerated holes are actually harvested and consumed by triethanolamine molecules on the surface of CdS NPs, generating oxidation product(s). Only a small amount of the photo-generated holes in the VB of CdS NPs is transferred to the VB of NiPS 3 UNSs (Fig. 7 ). In contrast, much more photogenerated electrons in the CB of CdS NPs are transported to the CB of NiPS 3 UNSs. As shown in Fig. 7 , four kinds of HER reactive sites are present on NiPS 3 : (1) P, S2 and S3 sites at (100) edge, (2) S site at (010) edge, (3) P1, S2, S3 and S8 sites at (1−30) edge and (4) activated S site at the basal plane. Hence, the photogenerated electrons could efficiently reduce the protons to evolve H 2 gas molecules at the above four kinds of highly active HER sites on NiPS 3 UNSs in NiPS 3 /CdS system. Therefore, this NiPS 3 /CdS heterojunction assures both efficient electron-hole dissociation/migration and boosts HER activity, thus leading to the highly enlarged photocatalytic H 2 production (Fig. 4a ). Additionally, since the enhanced visible-light absorption by NiPS 3 UNSs cannot contribute to the photocatalytic H 2 production, the light absorption and generation of photoinduced charge carriers by NiPS 3 UNSs are not depicted in Fig. 7 . This mechanism demonstrates that the type I heterojunction can also achieve highly efficient photocatalytic performance in some conditions. Fig. 7: Schematic illustration of photocatalytic H 2 -production mechanism in NiPS 3 /CdS system. The visible-light excitation ( λ > 400 nm), separation/migration of photogenerated electrons and holes, and the surface catalytic reactions of NiPS 3 /CdS system are shown in the figure. Full size image Generality of NiPS 3 UNSs To support the generality of NiPS 3 UNSs platform for advancing photocatalytic H 2 production, the other three systems were also explored. The XRD patterns of TiO 2 and NiPS 3 /TiO 2 (Supplementary Fig. 29a ), In 2 ZnS 4 and NiPS 3 /In 2 ZnS 4 (Supplementary Fig. 29b ), as well as C 3 N 4 and NiPS 3 /C 3 N 4 (Supplementary Fig. 29c ) are displayed in the supporting information. As shown in Supplementary Fig. 29a–c , no obvious alteration in the positions and intensities of diffraction peaks are observed on the patterns for hybrid samples (NiPS 3 /TiO 2 , NiPS 3 /In 2 ZnS 4 and NiPS 3 /C 3 N 4 ), in contrast to their pure counterparts (TiO 2 , In 2 ZnS 4 and C 3 N 4 ). These results indicate that the physical mixing process in the mortar at room temperature does not alter the crystal/phase structures of TiO 2 , In 2 ZnS 4 or C 3 N 4 . No diffraction peaks assigned to NiPS 3 UNSs are found on the XRD patterns of NiPS 3 /TiO 2 , NiPS 3 /In 2 ZnS 4 and NiPS 3 /C 3 N 4 (Supplementary Fig. 29a–c ), suggesting the homogenous dispersion and low amount of NiPS 3 UNSs in the merged samples (NiPS 3 /TiO 2 , NiPS 3 /In 2 ZnS 4 and NiPS 3 /C 3 N 4 ). The TEM images of NiPS 3 /TiO 2 (Supplementary Fig. 30a ), NiPS 3 /In 2 ZnS 4 (Supplementary Fig. 30b ) and NiPS 3 /C 3 N 4 (Supplementary Fig. 30c ), respectively, confirm the combination of NiPS 3 UNSs with TiO 2 NPs, In 2 ZnS 4 NSs and C 3 N 4 , respectively. Also, the HRTEM images (Supplementary Fig. 30d–f ) as well as the EDX spectra (Supplementary Fig. 30g–i ) further support the merging of NiPS 3 UNSs with TiO 2 NPs, In 2 ZnS 4 NSs and C 3 N 4, respectively. Moreover, the HAADF-STEM images and the corresponding elemental mapping images of NiPS 3 /TiO 2 (Supplementary Fig. 31a–f ), NiPS 3 /In 2 ZnS 4 (Supplementary Fig. 31g–l ) and NiPS 3 /C 3 N 4 (Supplementary Fig. 31m–r ) also support coupling of NiPS 3 UNSs with TiO 2 NPs, In 2 ZnS 4 NSs and C 3 N 4, respectively. The high-resolution XPS spectra of NiPS 3 /TiO 2 (Supplementary Fig. 17a–d ), NiPS 3 /In 2 ZnS 4 (Supplementary Fig. 17e–h ) and NiPS 3 /C 3 N 4 (Supplementary Fig. 17i–l ) confirm the intimate electronic coupling between NiPS 3 and TiO 2 , In 2 ZnS 4 , C 3 N 4 , respectively. The efficient charge separation and transport in NiPS 3 /TiO 2 , NiPS 3 /In 2 ZnS 4 and NiPS 3 /C 3 N 4 are supported by both the steady-state PL spectra in Supplementary Fig. 32a–c and transient-state PL spectra in Supplementary Fig. 32d–f . The data presented in Supplementary Fig. 32d–f insets also prove that all the fitting charge carrier lifetimes and intensity-averaged charge carrier lifetimes obtained for NiPS 3 /TiO 2 , NiPS 3 /In 2 ZnS 4 and NiPS 3 /C 3 N 4 are elongated after loading of NiPS 3 UNSs, compared to the bare counterparts, respectively. To study the intimate interaction in all the NiPS 3 -based samples, the Zeta potentials of NiPS 3 UNSs, TiO 2 NPs, CdS NPs, In 2 ZnS 4 NSs and C 3 N 4 in ethanol were acquired. As shown in Supplementary Fig. 33 , NiPS 3 UNSs, TiO 2 NPs, CdS NPs, In 2 ZnS 4 NSs and C 3 N 4 show the Zeta potentials of −2.73, −0.36, −57.3, −58 and 12.5 mV in ethanol, respectively. These results indicate the repulsive electrostatic forces between NiPS 3 UNSs and TiO 2 NPs, CdS NPs or In 2 ZnS 4 NSs. However, the TEM images (Fig. 2a and Supplementary Fig. 30a, b ) confirm the combination of NiPS 3 UNSs with TiO 2 NPs, CdS NPs and In 2 ZnS 4 NSs, respectively. And the XPS results (Fig. 3a and Supplementary Fig. 17a–h ) further indicate the electronic coupling between NiPS 3 UNSs and TiO 2 NPs, CdS NPs or In 2 ZnS 4 NSs. These results suggest that Van der Waals force rather than the electrostatic force should be the main force leading to the strong electronic coupling in NiPS 3 /CdS, NiPS 3 /TiO 2 and NiPS 3 /In 2 ZnS 4 systems. Furthermore, as for the NiPS 3 /C 3 N 4 system, the opposite Zeta potentials for NiPS 3 (−2.73 mV) and C 3 N 4 (12.5 mV) are observed in Supplementary Fig. 33 . Thus, the attractive electrostatic force and Van der Waals force together result in the strong coupling between NiPS 3 UNSs and C 3 N 4 , as evidenced by the TEM image (Supplementary Fig. 30c ) and XPS results (Supplementary Fig. 17i–l ). The electrochemical HER activities shown in Supplementary Fig. 34a–c further prove that the integration of NiPS 3 UNSs with TiO 2 NPs, In 2 ZnS 4 NSs and C 3 N 4 can greatly boost the HER activities. In addition, the UV-Vis diffuse reflectance spectra of TiO 2 and NiPS 3 /TiO 2 (Supplementary Fig. 35a ), In 2 ZnS 4 and NiPS 3 /In 2 ZnS 4 (Supplementary Fig. 35b ), as well as C 3 N 4 and NiPS 3 /C 3 N 4 (Supplementary Fig. 35c ) are also presented in supporting information. The addition of NiPS 3 UNSs leads to greatly improved visible-light absorption owing to the strong absorption of NiPS 3 with a small band gap ( E = 1.42 eV). However, under the illumination of 630-nm LED, NiPS 3 /TiO 2 , NiPS 3 /In 2 ZnS 4 and NiPS 3 /C 3 N 4 exhibit negligible photocatalytic H 2 -production activity (Supplementary Fig. 35d–f ), again suggesting that the increased light absorption caused by NiPS 3 UNSs does not contribute to the activity enhancement. The above-mentioned results strongly support the ability of NiPS 3 UNSs to efficiently improve the photocatalytic H 2 -production rates for different kinds of semiconductor photocatalysts, which demonstrates a huge potential of the emerging MPC x family in photocatalysis. This work shows that the edge of NiPS 3 UNSs possesses abundant atomic-level P/S active sites while the basal plane exhibits relatively lower HER activity. Although it is hard to selectively load the CdS NPs at the edge rather than the basal plane of NiPS 3 UNSs for achieving further activity improvement, NiPS 3 UNSs with smaller lateral sizes and more edge active sites can be synthesized to facilitate the loading of CdS NPs at/near the edge of NiPS 3 UNSs. This will be explored in our future study. In summary, we report for the first time a facile liquid exfoliation technique to synthesize the MPC x group of materials, 2D NiPS 3 , with an ultrathin thickness (~3.16 nm). The as-synthesized NiPS 3 UNSs serve as a universal platform to elevate the light-driven H 2 -production performance of various photocatalysts, including TiO 2 , CdS, In 2 ZnS 4 and C 3 N 4 . The as-prepared NiPS 3 /CdS hybrid displays the highest photocatalytic hydrogen (H 2 ) production activity (13,600 μmol h −1 g −1 ), with the largest enhancement factor of ~1667%, in contrast to that of pristine CdS. The greatly raised performance of NiPS 3 /CdS is due to two reasons: (1) the electronically coupled interfaces between NiPS 3 UNSs and CdS NPs apparently facilitate the charge-carrier separation/transport. Particularly, the transport of photogenerated holes to the surface of CdS NPs is significantly boosted, which are harvested by the sacrificial electron donor, triethanolamine. Thus, the remaining photogenerated electrons on CdS NPs could efficiently migrate to NiPS 3 UNSs for H 2 evolution; (2) numerous atomic-level P/S edge sites and activated S basal sites of NiPS 3 UNSs tremendously advance H 2 evolution reaction. These findings are supported by both theoretical computations and advanced characterizations, such as atomic-resolution AC-STEM, transient-state PL spectroscopy, transient-state SPV spectroscopy, ultrafast TAS and in situ XPS. Our study not only shows the great potential of MPC x family as a general platform to immensely increase the light-induced H 2 -production activities on various semiconductor photocatalysts but more importantly, shed light on the rational design/preparation of photocatalysts through understanding of the atomic-level structure/composition-activity correlation and electron-hole kinetics/thermodynamics in photocatalysis. Synthesis of NiPS 3 UNSs NiPS 3 UNSs were fabricated by a liquid exfoliation method. In detail, 50 mg of commercial bulk NiPS 3 powder (Ossila, UK) were ground into a fine powder and added to 50 mL of ethanol and ultrasonicated in an ice bath for 200 min. The resultant dispersion was centrifuged at 8000 RPM (6016 × g ) for 2 min and the supernatant was reserved for use. The concentration of NiPS 3 UNSs in ethanol solution was determined to be ~109.97 μg mL −1 using ICP-AES. Synthesis of CdS NPs CdS NPs were synthesized using a precipitation-hydrothermal technique. First, 3.424 g of Cd(NO 3 ) 2 ·4H 2 O were put into 87 mL of deionized water followed by stirring for 1 h. Then, 20 mL of 0.9 M Na 2 S aqueous solution were added dropwise into the above solution, followed by 1-h stirring. At last, the suspension was transferred to a 200 mL Teflon-lined autoclave and maintained at 180 °C for 12 h. The resulting products were washed with deionized water and ethanol twice, respectively, and dried at 60 °C for 300 min. CdS NPs were denoted as 0.0N. Synthesis of In 2 ZnS 4 nanosheets (NSs) In 2 ZnS 4 NSs were fabricated utilizing a hydrothermal method. Specifically, 0.277 g of Zn(NO 3 ) 2 ·6H 2 O, 0.560 g of In(NO 3 ) 3 · x H 2 O and 0.559 g of thioacetamide were put into 140 mL of deionized water with constant stirring. Afterward, 21.1 mL of 1.0 M HCl aqueous solution were added to the above aqueous solution. The resulting aqueous solution was transferred to a 200 mL hydrothermal autoclave and kept at 160 °C for 12 h. Synthesis of C 3 N 4 C 3 N 4 was synthesized via grinding 5 g of urea, 5 g of thiourea and 20 mg of Pluronic F127 and adding the resulting mixture into a crucible followed by heating at 350 °C for 1 h and 600 °C for 3 h. The as-synthesized sample was ground into fine powder. Synthesis of NiPS 3 /CdS heterojunction NiPS 3 /CdS heterostructure was synthesized by a self-assembly approach via mechanical mixing at room temperature. Specifically, 50 mg of the as-synthesized CdS NPs were put into the mortar, followed by adding 5.0, 10.0, 20.0 and 30.0 mL of NiPS 3 UNSs in ethanol, respectively. The suspension was then ground for 1 min. After evaporation of ethanol, the solid samples were finally ground to obtain fine powders and denoted as 5.0N, 10.0N, 20.0N and 30.0N, respectively. Synthesis of NiPS 3 /In 2 ZnS 4 heterojunction NiPS 3 /In 2 ZnS 4 heterostructure was fabricated using a self-assembly method through physical mixing at room temperature. In detail, 50 mg of the as-synthesized In 2 ZnS 4 NSs were added into the mortar followed by adding 20.0 mL of NiPS 3 UNSs in ethanol. The suspension was then ground for 1 min. After evaporation of ethanol, the solid sample was finally ground to a fine powder. Synthesis of NiPS 3 /TiO 2 heterojunction NiPS 3 /TiO 2 heterostructure was fabricated by a self-assembly method through mechanical mixing at room temperature. In detail, 50 mg of the as-synthesized Degussa P25 TiO 2 NPs were added into the mortar, followed by adding 20.0 mL of NiPS 3 UNSs in ethanol. The suspension was then ground for 1 min. After evaporation of ethanol, the solid sample was finally ground to obtain a fine powder. Synthesis of NiPS 3 /C 3 N 4 heterojunction NiPS 3 /C 3 N 4 heterojunction was synthesized by a self-assembly approach through mechanical mixing at room temperature. In detail, 50 mg of the as-synthesized C 3 N 4 were added into the mortar, followed by adding 20.0 mL of NiPS 3 UNSs in ethanol. The suspension was then ground for 1 min. After evaporation of ethanol, the solid sample was finally ground to obtain a fine powder. Physicochemical characterizations The XRD patterns of 0.0N, 5.0N, 10.0N, 20.0N, 30.0N and 20.0N-A were acquired on a silicon substrate on a powder X-ray diffractometer (D4 ENDEAVOR, Bruker) utilizing Co Kα radiation. The XRD patterns of In 2 ZnS 4 , NiPS 3 /In 2 ZnS 4 , TiO 2 , NiPS 3 /TiO 2 , C 3 N 4 and NiPS 3 /C 3 N 4 were obtained on a powder X-ray diffractometer (Miniflex, Rigaku) utilizing Cu Kα radiation. The FEI Themis Z double corrected S/TEM (Thermo Fisher Scientific, USA), FEI Titan S/TEM (Thermo Fisher Scientific, USA) and FEI tecani G2 Spirit TEM (Thermo Fisher Scientific, USA) were applied to acquire the TEM images, HRTEM images, EDS spectra, HAADF-STEM images, elemental mapping images and EELS spectra. A Multimode 8 (Bruker, USA) was used to obtain the AFM image and the height profile accordingly. The AFM profile was acquired after flattening treatment. An iHR550 Raman microscope (HORIBA scientific) with a charge-coupled device (CCD) detector and a confocal microscope were applied to acquire the Raman spectra. An Optima 8000 ICP-OES (Perkin Elmer, UK) was utilized to obtain the actual NiPS 3 amount in 20.0N sample. The in situ and ex-situ XPS measurements were performed on a K-Alpha plus XPS system (Thermo Fisher Scientific, USA). A light emitting diode was adopted as the light source to excite the photocatalysts in the in situ XPS measurements. A UV-Vis spectrophotometer (UV2600, Shimadzu, Japan) was utilized to obtain the UV-Vis diffuse reflectance spectra and UV-Vis absorption spectra. N 2 sorption analysis was conducted on a tristar II 3020 (Micromeritics, USA). A RF-5301PC spectrofluorophotometer (Shimadzu, Japan) was used to obtain the steady-state photoluminescence (PL) spectra at room temperature. A FLS1000 spectrometer (Edinburgh Instruments, UK) was utilized to acquire the transient-state PL spectra. The synchrotron radiation-based XANES measurements were performed at Hefei Synchrotron Radiation Facility (MCD-A and MCD-B Soochow Beamline for Energy Materials, NSRL) and XAS beamline in Australian Synchrotron (AS). A home-built apparatus introduced by Jing et al. [69] was used to acquire the steady-state SPV spectra. Another device described in the previous reference was adopted to obtain the transient-state SPV spectra. TAS used laser pulses sourced from the output of a Ti: sapphire regenerative amplifier (Spectra Physics, Spitfire Pro XP 100F), providing pulses centred at 800 nm with 100 fs duration and a 1 kHz repetition rate. The 400 nm excitation pulse was generated by frequency doubling of the fundamental output using a 0.5 mm BBO crystal. Pump-probe spectroscopic experiments were performed on a TA spectrometer (Ultrafast Systems, Helios). The 400 nm pump pulses had an energy of 0.1 μJ with a fwhm spot size of 350 μm, with a polarization rotated to the magic angle relative to the probe. The visible probe light was produced by focusing a small portion of the 800 nm amplifier output onto a 3.2 mm sapphire crystal. The white-light continuum was then split into signal and reference beams and focused onto the sample with a fwhm spot size of 100 μm. Samples were continuously stirred throughout the experiment, and photodegradation was <5%. The long-time TA spectra (up to 7.73 ns) were collected using a 400 nm laser with a power of 120 μW. The contact potential difference (CPD) test was measured on a Kelvin probe apparatus (Instytut Fotonowy, Poland) using the excitation light source of 427 nm. The Zeta potentials were acquired on a Zetasizer nano instrument (Malvern Panalytical, UK). Photocatalytic H 2 production test The photocatalytic H 2 -production test was performed in a 152 mL Pyrex flask with sealed silicone rubber septa at room temperature and atmospheric pressure. The light source is a 300 W xenon arc lamp with a UV-cutoff filter ( λ > 400 nm) for testing CdS-, In 2 ZnS 4 - and C 3 N 4 -based photocatalysts, and without any UV-cutoff filter for testing TiO 2 based photocatalysts. In a typical test, 20 mg of photocatalyst were added into 80 mL of ~17.0 vol% triethanolamine aqueous solution. Subsequently, ultrahigh purity Argon gas was purged into the suspension of photocatalyst for 30 min to remove air prior to illumination and make sure the anaerobic condition of the reactor. After that, 200 μL of gas were sampled intermittently through the septum followed by examining the generated H 2 on a gas chromatograph (Clarus 480, Perkin Elmer, USA) with a TDX-01 column and ultrahigh Argon as the carrier gas. Photocatalytic H 2 -production test using 630-nm LED was performed in the same conditions except that 300 W Xenon arc lamp was replaced by a 77 W 630-nm LED. The photocatalytic H 2 -production stability test of 20.0N in 0.35 M Na 2 S and 0.25 M Na 2 SO 3 aqueous solution was conducted in identical conditions except that ~17.0 vol% triethanolamine aqueous solution was replaced by the 0.35 M Na 2 S and 0.25 M Na 2 SO 3 aqueous solution. Apparent quantum yield test The apparent quantum yield (AQY) test was conducted in a top-irradiated 254 mL reactor using 70 mg 20.0N photocatalysts in 70 mL ~17.0 vol% triethanolamine aqueous solution. A 420-nm LED with a light intensity of 16.8 mW cm −2 was utilized as the light source. The AQY was calculated according to the following equation: 
    AQY (%)=	Reacted electron number/Incident photon number× 100 
    =	Generated _2 molecule number× 2/Incident photon number× 100
 (1) Electrochemical and photoelectrochemical measurements The Mott-Schottky plots were acquired using an electrochemical analyser (CHI760E instruments) in 0.5 M Na 2 SO 4 aqueous solution with a standard three-electrode system. Moreover, the identical three-electrode system was utilized to measure the TPC density in 0.5 M Na 2 SO 4 aqueous solution. A 300 W xenon light with a UV-cutoff filter ( λ > 400 nm) was utilized as the light source. 0.0N or 20.0N working electrode was prepared in a process as below: 10 mg of 0.0N or 20.0N, 15 mg of polyethylene glycol (PEG; molecular weight: 20,000) and 1.0 mL of ethanol were ground to produce a slurry. Then 0.1 mL of the slurry (equivalent to ~1 mg of 0.0N or 20.0N and 1.5 mg of PEG) was coated onto a 12 mm × 8 mm FTO glass electrode through a doctor-blade method. Finally, the coated electrode was dried and heated at 350 °C for 30 min with flowing ultrahigh purity argon flow. The NiPS 3 working electrode was synthesized as follows: 2 mL of NiPS 3 UNSs in ethanol (100 drops with 20 μL each time; equivalent to ~219.94 μg NiPS 3 UNSs) were dispersed onto the surface of a 12 mm × 8 mm FTO glass electrode. The acquired electrode was naturally dried in air and heated at 350 °C for 0.5 h under ultrahigh purity argon flow. Electrocatalyst ink was prepared by dispersing catalyst powder (2 mg) in a solution containing distilled water (Milli-Q, 482.5 μL), ethanol (482.5 μL) and 5 wt % Nafion solution (35 μL) followed by ultrasonication for 2 h. In all, 10 μL of catalyst ink was then deposited onto a polished glassy carbon electrode (diameter = 5 mm, area = 0.196 cm 2 , Pine Research Instrument). The mass loading of catalysts was determined as ~102 μg cm −2 . Electrochemical experiments were carried out using the rotating disk electrode method in a standard three-electrode glass cell at room temperature. A carbon rod was used as the counter electrode and an Ag/AgCl electrode (Pine Research Instrumentation) was used as the reference electrode. All potentials were converted to the reversible hydrogen electrode (RHE) and corrected with 95% iR-compensation. HER measurements were conducted in argon-saturated 0.1 M KOH electrolyte with a CHI potentiostat (CHI 760D) at a rotating speed of 1600 rpm. The polarization curves were recorded with a sweeping rate of 5 mV s −1 . The stability test was performed with 20 μL of catalyst ink deposited onto carbon paper (area = ~0.4 cm 2 , the mass loading of catalysts was ~100 μg cm −2 ) under a potential of −0.6 V vs. RHE. DFT calculations DFT calculations were applied to conduct all the electronic structure optimizations and calculations in this study. All the DFT calculations were conducted considering the solvation effect in 17 vol% triethanolamine aqueous solution using the VASPSOL, in which photocatalytic HER occurs. The Perdew–Burke–Ernzerhof (PBE) generalized gradient approximation (GGA) exchange–correlation functionals were applied using the projector-enhanced wave method through VASP software. Considering the solvent effect in 17% triethanolamine aqueous solution by volume, we set the dielectric constant of the solution to 29.36 and the Debye length to 2.68 Å. According to different cut-off energy tests, a plane wave cut-off energy of 520 eV was set, and the energy error is 0.01 eV. The convergence criteria for structural relaxation and energy calculation are: (1) self-consistent field energy tolerance is 1.0 × 10 -5 eV; (2) all the atoms in the systems were fully relaxed and maximum force tolerance on each atom is smaller than 0.05 eV Å −1 . During the geometry optimization and the total energy calculations, the smearing value was set as 0.2 eV. The approximate method developed by Grimme et al. [70] (zero damping DFT-D3 method of Grimme) was applied during all calculations to account for the contribution of the Van der Waals interactions between atoms to the energy. The structural optimization parameters for acquiring the hydrogen adsorption Gibbs free energy are displayed as follows: (i) (002) basal plane of NiPS 3 : unit cell parameters, a = 5.82 Å, b = 10.08 Å, c = 43.04 Å, α = 90º, β = 90º, γ = 90º, K -points setting of 5 × 3 × 1. (ii) (100) edge of NiPS 3 : unit cell parameters, a = 10.08 Å, b = 34.92 Å, c = 43.04 Å, α = 90º, β = 90º, γ = 90º, K -points setting of 3 × 1 × 1. (iii) (010) edge of NiPS 3 : unit cell parameters, a = 5.82 Å, b = 30.25 Å, c = 43.04 Å, α = 90º, β = 90º, γ = 90º, K -points setting of 5 × 1 × 1. (iv) (1−30) edge of NiPS 3: unit cell parameters, a = 6.90 Å, b = 15.40 Å, c = 33.65 Å, α = 79.33º, β = 94.87º, γ = 93.02º, K -points setting of 5 × 1 × 1. (v) NiPS 3 (002) facet/CdS (200) facet heterostructure: unit cell parameters, a = 5.84 Å, b = 10.91 Å, c = 57.25 Å, α = 90º, β = 90º, γ = 90º, K -points setting of 5 × 3 × 1. The structural optimization parameters for acquiring the work functions (Φ) are shown as follows: (i) (200) facet of CdS (space group F-43m): a = 5.86 Å, b = 11.73 Å, c = 50.26 Å, α = β = γ = 90º, K -points setting of 5 × 3 × 1. (ii) (002) facet of NiPS 3 (space group C2/m): a = 5.82 Å, b = 10.08 Å, c = 43.04 Å, α = β = γ = 90º, K -points setting of 5 × 3 × 1. The structural optimization parameters for acquiring the differential charge density map of NiPS 3 (002) facet/CdS (200) facet CdS heterostructure are shown as follows: a = 5.84 Å, b = 10.91 Å, c = 57.25 Å, α = 90º, β = 90º, γ = 90º, K -points setting of 5 × 3 × 1. The HSE06 hybrid functional was used to calculate the band structures and DOS of CdS (200) facet and NiPS 3 . The plane wave cut-off energy of 520 eV was set, and the energy error is 0.01 eV. The self-consistent field energy tolerance is 1.0 × 10 −5 eV. The calculation path of CdS (200) facet band structure is G-X-M-G, and the numbers of K -points are 17, 8 and 20. The calculation path of NiPS 3 band structure is G-M-K-G, and the numbers of K -points are 15, 8 and 17. The lattice parameters of CdS (200) facet and NiPS 3 are as follows: (i) CdS (200) facet, a = 5.86 Å, b = 11.73 Å, c = 21.46 Å, α = β = γ = 90º. (ii) NiPS 3 , a = 5.82 Å, b = 5.82 Å, c = 26.28 Å, α = β = 90º, γ = 120.02º. The atomic coordinates of the above structures are displayed in Supplementary Tables 13 – 18 .